A reasonable approach for the generation of hollow icosahedral kernels in metal nanoclusters Although the hollow icosahedral M 12 kernel has been extensively observed in metal nanoclusters, its origin remains a mystery. Here we report a reasonable avenue for the generation of the hollow icosahedron: the kernel collapse from several small nano-building blocks to an integrated hollow icosahedron. On the basis of the Au alloying processes from Ag 28 Cu 12 (SR) 24 to the template-maintained Au x Ag 28-x Cu 12 (SR) 24 and then to the template-transformed Au 12 Cu y Ag 32-y (SR) 30 , the kernel evolution/collapse from “tetrahedral Ag 4 + 4 ∗ Ag 3 ” to “tetrahedral Au 4 + 4 ∗ M 3 (M = Au/Ag)” and then to “hollow icosahedral Au 12 ” is mapped out. Significantly, the “kernel collapse” from small-sized nano-building blocks to large-sized nanostructures not only unveils the formation of hollow icosahedral M 12 in this work, but also might be a very common approach in constructing metallic kernels of nanoclusters and nanoparticles (not limited to the M 12 structure). Metal nanoclusters are an emerging class of modular nanomaterials [1] , [2] , [3] , [4] , [5] , [6] , and have been sparking great research interests owing to their atomically precise structures and intriguing properties [7] , [8] , [9] , [10] , [11] , [12] , [13] , [14] , [15] , [16] , [17] , [18] , [19] , [20] , [21] , [22] , [23] , [24] , [25] , [26] , [27] . The physiochemical properties of these nanomaterials, such as chirality, luminescence, catalysis, magnetism, and electrochemistry, can be rationalized in terms of their quantum size effect as well as discrete electronic states [28] , [29] , [30] , [31] , [32] , [33] , [34] , [35] , [36] , [37] , [38] . Besides, the atomically precise nature of these modular nanomaterials is of the most interest — indeed, compared with large-sized nanoparticles, nanoclusters (typically <2 nm of the metallic kernel) present more precise compositions/constructions, and thus allow for the atomic-level elucidation of structural evolutions and structure-property correlations [1] , [2] , [3] , [4] , [5] , [6] , [39] , [40] , [41] , [42] , [43] , [44] , [45] , [46] . Of all reported nanoclusters with precise structures, the icosahedral configuration is the most typical, which is frequently observed in both metal kernels and ligand shells of nanoclusters [47] , [48] , [49] , [50] , [51] . Interestingly, except for the non-hollow icosahedral M 1 @M 12 kernel (M represents the metal), the hollow icosahedral M 12 kernel has also served as a basic nano-building block of nanoclusters (e.g., Ag 44 (SR) 30 , Au 12+ n Cu 32 (SR) 30+ n , Ag 50 (dppm) 6 (SR) 30 , Au 144 (SR) 60 , etc.) [10] , [11] , [52] , [53] , [54] , [55] , [56] . Structurally, it is accepted that the non-hollow icosahedron might be more energetically favorable than the corresponding hollow one due to the extra 12 metal···metal interactions in M 1 @M 12 ; accordingly, the hollow icosahedral kernel is unlikely to arise in the initial stage of the nanocluster growth. Besides, the hollow M 12 kernel is also less likely to originate from its non-hollow counterpart because the 12 metal···metal interactions make it difficult to extract the innermost metal atom out. In this context, the origin of such hollow icosahedral kernels remains a mystery. In this work, based on the Au-alloying-induced nanocluster transformation from M 40 (SR) 24 to M 44 (SR) 30 (M = Au/Ag/Cu), a reasonable avenue for the generation of hollow icosahedral M 12 kernels has been mapped out, i.e., the kernel collapse from several small nano-building blocks to an integrated hollow icosahedron. The proposed avenue might serve as a common approach in constructing metallic kernels of nanoclusters and nanoparticles (not limited to the M 12 structure). Structural anatomy of M 40 (SR) 24 and M 44 (SR) 30 nanoclusters For the clarity of the structural transformation and the corresponding kernel collapse, the nanocluster structures involved in this work are first discussed (Fig. 1 ) — (i) M 40 (SR) 24 (M = Au/Ag/Cu; SR = SPhCl 2 ): the M 40 (SR) 24 nanoclusters start from the bi-metallic Ag 28 Cu 12 (SR) 24 [57] . 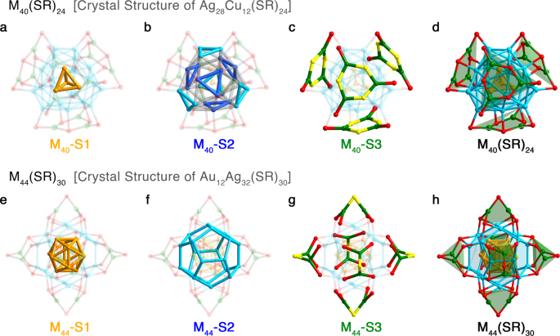Fig. 1: Structure anatomies of M40(SPhCl2)24and M44(SPhCl2)30(M = Au/Ag/Cu). a–dStructure anatomy of M40(SPhCl2)24:aM40-S1: the tetrahedral M4kernel;bM40-S2: the M24shell;cM40-S3: the Cu12(SR)24surface; anddThe overall structure of M40(SPhCl2)24.e–hStructure anatomy of M44(SPhCl2)30.eM44-S1: the hollow icosahedral M12kernel;fM44-S2: the M20shell;gM40-S3: the M12(SR)30surface; andhThe overall structure of M44(SPhCl2)30. Color labels: orange/light blue/blue/green, Ag or Cu atoms at different positions; red, S. All C and H atoms are omitted for clarity. Figure 1a–d depict the structure anatomy of Ag 28 Cu 12 (SR) 24 . Ag 28 Cu 12 (SR) 24 adopts a three-shell configuration, in a form of Ag 4 (M 40 -S1)@Ag 24 (M 40 -S2)@4*Cu 3 (SR) 6 (M 40 -S3). The innermost Ag 4 is in tetrahedral (Fig. 1a ). The 24 Ag atoms on M 40 -S2 can be divided into two categories, and each of 12 Ag atoms constitute four Ag 3 triangles (Fig. 1b ). The Ag atoms highlighted in dark blue connect with inward SR ligands on M 40 -S3 (Fig. 1c , highlighted in yellow); in contrast, the Ag atoms in light blue links outward SR ligands (highlighted in red) on M 40 -S3. (ii) M 44 (SR) 30 (M = Au/Ag/Cu; SR = SPhCl 2 ): the Au 12 Ag 32 (SR) 30 nanocluster is adopted to analyze the structure of M 44 (SR) 30 [58] . Au 12 Ag 32 (SR) 30 also has a three-shell configuration: Au 12 (M 44 -S1)@Ag 20 (M 44 -S2)@6*Ag 2 (SR) 5 (M 44 -S3). Of note, the Au 12 kernel is a hollow icosahedron (Fig. 1e ). Fig. 1: Structure anatomies of M 40 (SPhCl 2 ) 24 and M 44 (SPhCl 2 ) 30 (M = Au/Ag/Cu). a – d Structure anatomy of M 40 (SPhCl 2 ) 24 : a M 40 -S1: the tetrahedral M 4 kernel; b M 40 -S2: the M 24 shell; c M 40 -S3: the Cu 12 (SR) 24 surface; and d The overall structure of M 40 (SPhCl 2 ) 24 . e – h Structure anatomy of M 44 (SPhCl 2 ) 30 . e M 44 -S1: the hollow icosahedral M 12 kernel; f M 44 -S2: the M 20 shell; g M 40 -S3: the M 12 (SR) 30 surface; and h The overall structure of M 44 (SPhCl 2 ) 30 . Color labels: orange/light blue/blue/green, Ag or Cu atoms at different positions; red, S. All C and H atoms are omitted for clarity. Full size image Au-alloying-induced transformation from M 40 (SR) 24 to M 44 (SR) 30 The Au-alloying structural transformation started from the bi-metallic Ag 28 Cu 12 (SR) 24 (Fig. 2 ). The slight Au alloying on Ag 28 Cu 12 (SR) 24 resulted in a tri-metallic Au x Ag 28- x Cu 12 (SR) 24 ( x = 1.32) nanocluster, wherein the tetrahedral Ag 4 kernel of Ag 28 Cu 12 (SR) 24 was partially alloyed by the incorporated Au (Fig. 2 and Supplementary Fig. 1 ). When more Au heteroatoms were doped into M 40 (SR) 24 (Au x Ag 28- x Cu 12 (SR) 24 , x = 7.56; Fig. 2 ), all sites of the tetrahedron were entirely occupied by Au; besides, the redundant Au heteroatoms were further arranged onto M 40 -S2, invading the Ag sites that related to outward SR thiols (light blue triangles in Fig. 1b and Supplementary Figs. 2 – 3 ). Of note, throughout the abovementioned Au-alloying processes the M 40 (SR) 24 framework retained. Furthermore, the overdose of Au heteroatom induced the structural transformation from M 40 (SR) 24 to M 44 (SR) 30 . Structurally, from the crystal structure of Au 12 Cu y Ag 32- y (SR) 30 ( y = 0–6; Avg. 3.74; Fig. 2 and Supplementary Fig. 4 ), the M 44 (SR) 30 nanocluster reached its stable state when Cu atoms only occupied the M 44 -S3. The corresponding bond lengths in M 40 (SR) 24 (including Ag 28 Cu 12 (SR) 24 , Au x Ag 28- x Cu 12 (SR) 24 ( x = 1.32), Au x Ag 28- x Cu 12 (SR) 24 ( x = 7.56), and Au 4 Ag 24 Cu 12 (SR) 24 ) or M 44 (SR) 30 (including Au 12 Ag 32 (SR) 30 and Au 12 Cu y Ag 32- y (SR) 30 , y = 3.74) nanoclusters were compared in detail (Supplementary Figs. 5 – 6 and Supplementary Tables 1 – 2 ). Fig. 2: Illustration of Au-alloying-induced structural evolution. Step I contains the Au-doping processes from Ag 28 Cu 12 (SR) 24 to Au x Ag 28- x Cu 12 (SR) 24 ( x = 1.32) and then to Au x Ag 28- x Cu 12 (SR) 24 ( x = 7.56), in which processes the M 40 (SR) 24 framework retains. Step II is the Au-doping process from Au x Ag 28- x Cu 12 (SR) 24 ( x = 7.56) to Au 12 Cu y Ag 32- y (SR) 30 ( y = 3.74), in which process the M 40 (SR) 24 framework transforms into M 44 (SR) 30 (M = Au/Ag/Cu). The Au proportion gradually increases with the nanocluater evolution from Ag 28 Cu 12 (SR) 24 to Au x Ag 28- x Cu 12 (SR) 24 ( x = 1.32), Au x Ag 28- x Cu 12 (SR) 24 ( x = 7.56), and Au 12 Cu y Ag 32- y (SR) 30 ( y = 3.74). Color labels: light blue, Ag; orange, Au; green, Cu; red, S. All C and H atoms are omitted for clarity. Full size image Despite our repeated best efforts to obtain the crystal structure of Au 12 Cu y Ag 32- y (SR) 30 , its perfect crystal data remains unavailable. Herein, for acquiring an excellent crystal data of Au 12 Cu y Ag 32- y (SR) 30 , we promoted the co-crystallization between the M 44 (SR) 30 and a small-sized M 40 (SR) 24 nanoclusters (Supplementary Figs. 7 – 9 ). Fortunately, the structures of both two nanoclusters were excellently determined (Au 4 Ag 24 Cu 12 (SR) 24 and Au 12 Cu y Ag 32- y (SR) 30 ( y = 3.74)) although both displayed strongly negative valence state (i.e., “−4”). In this context, the presence of (PPh 4 ) + cations neutralized the electrostatic repulsion between these clusters (Supplementary Fig. 8 ) and thus promoted the nanocluster co-crystallization, which was different from previously reported co-crystallized nanocluster cases with both “0” or opposite valence states [59] , [60] , [61] , [62] . In the crystal lattice of the co-crystallized nanoclusters, three types of nanoclusters were observed (Supplementary Fig. 7 ) — L -Au 4 Ag 24 Cu 12 (SR) 24 (A α , A β ), R -Au 4 Ag 24 Cu 12 (SR) 24 (B α , B β ), and Au 12 Cu y Ag 32- y (SR) 30 ( y = 3.74; C α , C β ), among which the α - and β -nanoclusters were identical, but arranged in different rotation angles (Supplementary Fig. 7a–c ). In contrast to the crystallization of homogeneous nanoclusters, which are typically packed into superlattices with simple translational symmetry, such as ABAB or ABCABC packing pattern [40] , the (AuAgCu) 40 and (AuAgCu) 44 nanoclusters were packed with a more complex pattern (Supplementary Fig. 7d–f ). From the x -axis view, the clusters were packed with an A α -B α -C α #A β -B β -C β pattern. α - and β -nanoclusters were arranged separately along the z -direction, giving rise to α - and β -cluster lines (Supplementary Fig. 7f ). In either cluster line, the adjacent three nanoclusters constituted a repetitive unit, A α -B α -C α or A β -B β -C β , which was labeled by red or black frames, respectively. Such repetitive units were also observed from y -axis and z -axis views (Supplementary Fig. 7 ). The optical absorptions of the obtained nanocluster crystals (dissolved in CH 2 Cl 2 ) were compared (Supplementary Fig. 10 ). Along with the Au-alloying process from Ag 28 Cu 12 (SR) 24 to Au x Ag 28- x Cu 12 (SR) 24 ( x = 1.32) and Au x Ag 28- x Cu 12 (SR) 24 ( x = 7.56), there was no significant alteration of the optical absorptions (405, 465, and 555 nm). By contrast, when the nanocluster template transformed from M 40 (SR) 24 to M 44 (SR) 30 , these absorptions shifted to 390, 490, and 595 nm immediately (Supplementary Fig. 10 ), demonstrating the remarkable change over electronic structures with the template transformation. Time-dependent UV-vis of the transformation from Ag 28 Cu 12 (SR) 24 to Au x Ag 28- x Cu 12 (SR) 24 and then to Au 12 Cu y Ag 32- y (SR) 30 were performed to track the cluster transformation (Supplementary Fig. 11a ). The changes of UV-vis contained two stages: (stage 1, from Ag 28 Cu 12 (SR) 24 to Au x Ag 28- x Cu 12 (SR) 24 ) eight isoabsorption points at 360, 385, 420, 445, 485, 550, 570, and 640 nm were observed (Supplementary Fig. 11b ); (stage 2, from Au x Ag 28- x Cu 12 (SR) 24 to Au 12 Cu y Ag 32- y (SR) 30 ) three isoabsorption points at 400, 485, and 510 nm were detected (Supplementary Fig. 11c ). The observation of these isoabsorption points suggested that the overall cluster transformation was a proportional conversion. Accordingly, both transformations from Ag 28 Cu 12 (SR) 24 to Au x Ag 28- x Cu 12 (SR) 24 and from Au x Ag 28- x Cu 12 (SR) 24 to Au 12 Cu y Ag 32- y (SR) 30 followed an “intramolecular rearrangement” approach, but not an “intermolecular decomposition-recombination” approach. Besides, along with the Au-alloying process, the thermal stability of nanoclusters was enhanced. As shown in Supplementary Fig. 12 , UV-vis characteristic absorptions of the Ag 28 Cu 12 (SR) 24 nanocluster (dissolved in CH 2 Cl 2 ) gradually decreased in intensity after 1 h and completely disappeared in ~4 h, indicating degradation. In contrast, the UV-vis absorptions of Au x Ag 28- x Cu 12 (SR) 24 ( x = 1.32) were essentially identical in the first 2 h, and gradually decreased as time went on. 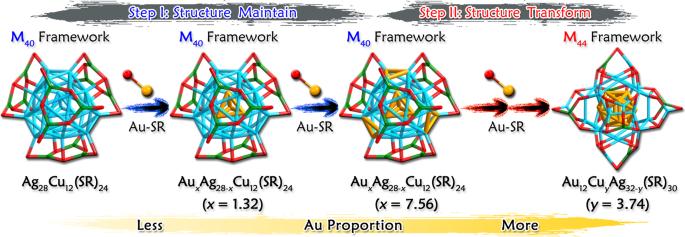Fig. 2: Illustration of Au-alloying-induced structural evolution. Step I contains the Au-doping processes from Ag28Cu12(SR)24to AuxAg28-xCu12(SR)24(x= 1.32) and then to AuxAg28-xCu12(SR)24(x= 7.56), in which processes the M40(SR)24framework retains. Step II is the Au-doping process from AuxAg28-xCu12(SR)24(x= 7.56) to Au12CuyAg32-y(SR)30(y= 3.74), in which process the M40(SR)24framework transforms into M44(SR)30(M = Au/Ag/Cu). The Au proportion gradually increases with the nanocluater evolution from Ag28Cu12(SR)24to AuxAg28-xCu12(SR)24(x= 1.32), AuxAg28-xCu12(SR)24(x= 7.56), and Au12CuyAg32-y(SR)30(y= 3.74). Color labels: light blue, Ag; orange, Au; green, Cu; red, S. All C and H atoms are omitted for clarity. Of note, the optical absorptions of Au x Ag 28- x Cu 12 (SR) 24 ( x = 7.56) was almost retained within 24 h, suggesting the enhanced thermal stability of Au x Ag 28- x Cu 12 (SR) 24 ( x = 7.56) over other two M 40 (SR) 24 nanoclusters. In this context, the sequence of the thermal stability of these three M 40 (SR) 24 nanoclusters was determined as Au x Ag 28- x Cu 12 (SR) 24 ( x = 7.56) > Au x Ag 28- x Cu 12 (SR) 24 ( x = 1.32) > Ag 28 Cu 12 (SR) 24 ; that is, increasing the Au-doping amount in nanoclusters was in favor of preparing M 40 (SR) 24 with higher thermal stability. Electrospray ionization mass spectrometry (ESI-MS) was then performed on nanocluster crystals (dissolved in CH 2 Cl 2 ), and the mass results confirmed the compositions of these “−4”-charged M 40 (SR) 24 and M 44 (SR) 30 nanoclusters (Supplementary Fig. 13 ). Besides, the in-situ Au-alloying process and the nanocluster template transformation were tracked by exploiting the ESI-MS (Supplementary Figs. 14 – 18 ). At the very beginning process (1–2 min in Supplementary Fig. 14 ), only Au x Ag 28- x Cu 12 (SR) 24 nanoclusters were detected (Fig. 2 ), corresponding to the Au-doping process from Ag 28 Cu 12 (SR) 24 to Au x Ag 28- x Cu 12 (SR) 24 ( x = 1.32) and Au x Ag 28- x Cu 12 (SR) 24 ( x = 7.56). The further Au-alloying induced both the Au component growth in M 40 (SR) 24 and the template transformation from M 40 (SR) 24 to M 44 (SR) 30 (3–6 min in Supplementary Fig. 14 ). Finally, only Au 12 Cu y Ag 32- y (SR) 30 nanoclusters could be observed (7–8 min in Supplementary Fig. 14 ), which suggested the complete transformation of nanoclusters. Of note, the Au 12 Ag 32- y Cu y (SR) 30 would stable at y = 3 or 4 once generated, matching with the crystal structure of Au 12 Cu y Ag 32- y (SR) 30 ( y = 3.74). Energy-dispersive X-ray spectroscopy (EDS) mapping and X-ray photoelectron spectroscopy (XPS) were conducted to confirm the Au-alloying process (Supplementary Figs. 19 – 28 ). 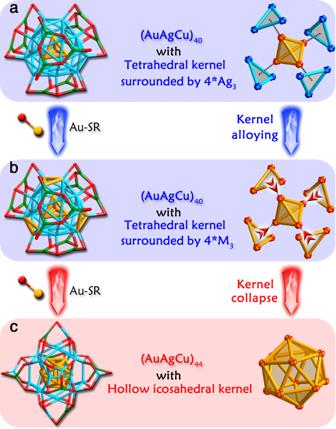Fig. 3: Kernel transformation from tetrahedron to hollow icosahedron. aCrystal structure of AuxAg28-xCu12(SR)24(x= 1.32) and its tetrahedral M4(M = Au/Ag) kernel surrounded by four Ag3triangles.bCrystal structure of AuxAg28-xCu12(SR)24(x= 7.56) and its tetrahedral Au4kernel surrounded by four M3(M = Au/Ag) triangles. The red arrows represent the trend of kernel collapse from “tetrahedral Au4+ 4∗M3” to “hollow icosahedral Au12”.cCrystal structure of Au12CuyAg32-y(SR)30(y= 3.74) and its hollow icosahedral Au12kernel. Color labels: light blue, Ag; orange, Au; green, Cu; red, S. All C and H atoms are omitted for clarity. Kernel transformation from tetrahedron to hollow icosahedron Figure 3 depicts the kernel collapse from the “tetrahedral Au 4 + 4*M 3 ” to “hollow icosahedral Au 12 ” induced by the Au alloying. Specifically, the initial Au-doping process transported the Au heteroatoms to the tetrahedral kernel, converting the Ag 4 kernel to the alloyed Au x Ag 4- x and the final Au 4 (Fig. 3a ). The further Au-alloying sites on M 40 -S2 predominantly located at the four M 3 triangles that adhered to a vertex-to-face relationship to the tetrahedral Au 4 kernel (Fig. 3b and Supplementary Fig. 3c ); in contrast, the other four triangles on M 40 -S2, following a face-to-face relationship to the Au 4 tetrahedral kernel, maintained unalloyed as Ag 3 (Supplementary Fig. 3d ). For easily distinguishing these M 3 positions, we define these Au 3 positions as “stable location” (Supplementary Fig. 3c ) and “unstable location” (Supplementary Fig. 3d ). However, the Au doping on stable locations is simply concluded from the crystallography, and the Au positions may change throughout the crystallization process. From ESI-MS results (Supplementary Fig. 14 ), a maximum of 18–19 Au heteroatoms could be doped into the M 40 cluster framework, >16 positions from the M 4 kernel and 4*M 3 stable locations; accordingly, there are other Ag positions in M 40 that could be occupied by the introduced Au. X-ray absorption fine structure spectroscopy (XAFS) measurements were then performed for grasping the in-situ Au-doping process (Supplementary Figs. 29 and 30 and Supplementary Tables 3 – 4 ). The XAFS results demonstrated that the introduced Au occupied the innermost M 4 tetrahedron first, and then substituted the Ag atoms in unstable locations, different from the crystal results wherein the unstable locations were maintained as undoped Ag throughout. We further crystallized this cluster sample and the crystal data suggested the Au heteroatoms on stable locations (i.e., Au x Ag 28- x Cu 12 (SR) 24 , x = 7.76), demonstrating the intracluster Au–Ag metal exchange throughout the crystallization. In this context, we made some speculations on mass signals (Supplementary Fig. 14 ): the introduced Au heteroatoms occupied the innermost tetrahedron first, and then substituted Ag atoms on M 40 -S2 randomly; the mass signals i represented the dominant Au-occupation in stable locations, whereas the signals ii represented the unstable locations, resulting in two groups of signals in the 3-min mass spectrum (Supplementary Fig. 14 ). In the 3-min sample, the M 40 with Au-occupation in unstable locations might be the main product by referring XAFS results. Then, the M 40 clusters of signals ii would transform to M 44 clusters of signals iii, and then decomposed due to their instability. By comparison, the M 40 clusters of signals i were continually doped by Au and transformed to M 44 clusters of signals iv finally. In this context, the driving force for the transformation from M 40 to M 44 was determined as the Au-alloying at unstable locations, which rendered the M 40 nanoclusters unstable molecules and triggered the kernel collapse from several small nano-building blocks to an integrated hollow icosahedron. Fig. 3: Kernel transformation from tetrahedron to hollow icosahedron. a Crystal structure of Au x Ag 28- x Cu 12 (SR) 24 ( x = 1.32) and its tetrahedral M 4 (M = Au/Ag) kernel surrounded by four Ag 3 triangles. b Crystal structure of Au x Ag 28- x Cu 12 (SR) 24 ( x = 7.56) and its tetrahedral Au 4 kernel surrounded by four M 3 (M = Au/Ag) triangles. The red arrows represent the trend of kernel collapse from “tetrahedral Au 4 + 4 ∗ M 3 ” to “hollow icosahedral Au 12 ”. c Crystal structure of Au 12 Cu y Ag 32- y (SR) 30 ( y = 3.74) and its hollow icosahedral Au 12 kernel. Color labels: light blue, Ag; orange, Au; green, Cu; red, S. All C and H atoms are omitted for clarity. Full size image Significantly, the further Au-alloying induced the transformation from M 40 (SR) 24 to M 44 (SR) 30 , among which process the hollow icosahedral Au 12 was generated (Fig. 3b, c ). Structurally, the pre-transformed Au x Ag 28- x Cu 12 (SR) 24 possesses a “tetrahedral Au 4 + 4*M 3 ” kernel (M = Au/Ag with a high Au proportion). Upon the nanocluster conversion, the M 3 triangles collapsed inward to the Au 4 tetrahedron, and finally rearranged into the hollow icosahedral Au 12 kernel in Au 12 Cu y Ag 32- y (SR) 30 (Fig. 3c ). Of note, there are 16 metal atoms in the “tetrahedral M 4 + 4*M 3 ” kernel while the icosahedral kernel only contains 12 metal atoms; in this context, a structural rearrangement occurred in this structural and kernel transformation (indeed, the “kernel+surface” configurations between M 40 (SR) 24 and M 44 (SR) 30 nanoclusters are different). However, due to the existence of several isoabsorption points in the UV-vis spectra, the structure transformation from M 40 (SR) 24 to M 44 (SR) 30 should follow an “intramolecular rearrangement” approach, but not an “intermolecular decomposition-recombination” approach. Accordingly, it is reasonable to conjecture the formation of icosahedral M 12 in M 44 (SR) 30 as the kernel collapse from “tetrahedral Au 4 + 4*M 3 ”. Besides, all sites in the hollow icosahedron are fully occupied by Au (i.e., Au 12 ); in vivid contrast, the non-hollow M 1 @M 12 kernels of previously alloy clusters are always partially occupied by two or more types of metals. We proposed that the complete Au occupation of the hollow icosahedron resulted from the kernel collapse in which process only the collapse of Au atom to Au 4 was the most energetically favorable. This avenue (i.e., kernel collapse) is of great importance since it maps out a reasonable avenue for the generation of the hollow icosahedral M 12 kernel in metal nanoclusters. Besides, the kernel collapse might be a very common approach in constructing metallic kernels of nanoclusters and nanoparticles (not limited to the hollow icosahedron, but also compliant to other configurations such as non-hollow icosahedron, FCC/BCC kernels, etc. ), because the routine growth of several large-sized nanoclusters shell-by-shell should be not that energetically favorable. We also note that the kernel collapse should not be the unique approach for the generation of hollow icosahedra (or other structures) in metal nanoclusters and nanoparticles; other approaches may also exist and are still worth mapping out. In summary, on the basis of the Au-alloying-induced transformation from M 40 (SR) 24 to M 44 (SR) 30 (M = Au/Ag/Cu), a reasonable avenue—kernel collapse—for the generation of the hollow icosahedral M 12 kernel in metal nanoclusters has been mapped out. The Au alloying on Ag 28 Cu 12 (SR) 24 produced template-maintained Au x Ag 28- x Cu 12 (SR) 24 ( x = 1.32), Au x Ag 28- x Cu 12 (SR) 24 ( x = 7.56), and template-transformed Au 12 Cu y Ag 32- y (SR) 30 ( y = 3.74) step by step, accompanying with which processes the cluster kernel stepwisely evolved from “tetrahedral Ag 4 + 4*Ag 3 ” to “tetrahedral Au 4 + 4*Ag 3 ”, then to “tetrahedral Au 4 + 4*Au 3 ”, and finally to “hollow icosahedral Au 12 ”. The entire process was tracked by ESI-MS, and the crystal structures of the key nodes (altogether five crystal structures) have been determined. Overall, this work presents a reasonable avenue for comprehending the generation of hollow icosahedra in metal nanoclusters, and the “structure collapse” might be a very common approach for constructing kernel structures (not limited to the hollow icosahedron) in the size growth of nanoclusters and nanoparticles. Materials All reagents were purchased from Sigma-Aldrich and used without further purification: silver nitrate (AgNO 3 , 99%, metal basis), tetrachloroauric (III) acid (HAuCl 4 ·3H 2 O, 99.99% metal basis), copper(II) acetylacetonate (Cu(O 2 C 5 H 7 ) 2 , 99%, metal basis), 2,4-dichlorobenzenethiol (HSPhCl 2 , 99%), sodium borohydride (NaBH 4 , 97%), tetraphenylphosphonium bromide ((PPh 4 )Br, 95%), dichloromethane (CH 2 Cl 2 , HPLC, Sigma-Aldrich), methanol (CH 3 OH, HPLC, Sigma-Aldrich), N,N-dimethylformamide (DMF, HPLC, Sigma-Aldrich), hexane (C 6 H 6 , HPLC, Sigma-Aldrich), and ethyl ether ((CH 3 CH 2 )O, HPLC, Sigma-Aldrich). Synthesis of Au(I)-SPhCl 2 For the Au(I)-SPhCl 2 complexes synthesis, HAuCl 4 ·3H 2 O (1 mmol) was dissolved in 5 mL CH 3 OH, and 2,4-dichlorobenzenethiol (500 μL, 4 mmol) was dissolved in 5 mL CH 3 OH and added drop-wise to the solution under vigorously stirring (~1200 rpm). After reacted for 15 min, the resulting precipitate was washed several times with hexane. Then the final product was used directly. Synthesis of [Ag 28 Cu 12 (SPhCl 2 ) 24 ] 4− The Ag 28 Cu 12 (SPhCl 2 ) 24 was prepared by a literature method reported by the Zheng group with some modification [57] . Specifically, 60 mg of Cu(O 2 C 5 H 7 ) 2 was dissolved in 5 mL of CH 3 OH and 15 mL of CH 2 Cl 2 , to which 60 mg AgNO 3 (dissolved in 2 mL of H 2 O) was added. After stirring for 20 min, 100 μL of HSPhCl 2 was added in, and the reaction further processed for 30 min. Then, 30 mg NaBH 4 (dissolved in 2 mL of H 2 O) was added in. The reaction was allowed to proceed for 5 h. After that, the aqueous layer was removed, and the mixture in the organic phase was rotavaporated under vacuum. Then 50 mL of CH 3 OH was used to extract the Ag 28 Cu 12 (SPhCl 2 ) 24 nanocluster, to which supernatant 20 mg of (PPh 4 )Br was added in. The precipitate was then washed three times by CH 3 OH. Then the final product, i.e., [Ag 28 Cu 12 (SPhCl 2 ) 24 ] 4− (PPh 4 ) 4 , was used directly. The yield is 35% based on the Ag element (calculated from the AgNO 3 ). Syntheses of [Au x Ag 28- x Cu 12 (SPhCl 2 ) 24 ] 4− (x = 1.32), [Au x Ag 28- x Cu 12 (SPhCl 2 ) 24 ] 4− ( x = 7.56), and [Au 12 Cu y Ag 32- y (SPhCl 2 ) 30 ] 4− nanoclusters These three nanoclusters were prepared from parallel Au-alloying reactions (in the same condition but were stopped at different times). Specifically, 20 mg of Ag 28 Cu 12 (SPhCl 2 ) 24 was first dissolved in 20 mL of CH 2 Cl 2 and then 5 mg of Au(I)-SPhCl 2 complexes was added in. After 2 min, 100 mL of hexane was poured in to pause the reaction; the precipitate was then dissolved in 20 mL of CH 2 Cl 2 to yield the Au x Ag 28- x Cu 12 (SPhCl 2 ) 24 ( x = 1.32). Expanding the reaction time from 2 min to 3 min would produce the Au x Ag 28- x Cu 12 (SPhCl 2 ) 24 ( x = 7.56). Expanding the reaction time from 2 min to 8 min would produce the Au 12 Cu y Ag 32- y (SPhCl 2 ) 30 . Synthesis of [Au 12 Ag 32 (SPhCl 2 ) 30 ] 4− The Au 12 Ag 32 (SPhCl 2 ) 30 nanocluster was prepared by a literature method reported by the Zheng group [58] . Preparation of XAFS samples In all, 10 mg of Ag 28 Cu 12 (SPhCl 2 ) 24 was dissolved in 10 mL of CH 2 Cl 2 and then 3 mg of Au(I)-SPhCl 2 complexes was added in. After 1 min, 200 mL of hexane was poured in to pause the reaction; the precipitate was then dissolved in 5 mL of CH 2 Cl 2 to yield the Au x Ag 28- x Cu 12 (SPhCl 2 ) 24 (Sample 1). In total, 10 mg of Ag 28 Cu 12 (SPhCl 2 ) 24 was first dissolved in 10 mL of CH 2 Cl 2 and then 3 mg of Au(I)-SPhCl 2 complexes was added in. After 2 min, 200 mL of hexane was poured in to pause the reaction; the precipitate was then dissolved in 5 mL of CH 2 Cl 2 to yield the Au x Ag 28- x Cu 12 (SPhCl 2 ) 24 (Sample 2). Single crystals of XAFS Sample 2 (i.e., Au x Ag 28- x Cu 12 (SPhCl 2 ) 24 , x = 7.76) were cultivated at room temperature by vapor diffusing the ethyl ether into the DMF solution of nanoclusters. Crystallization of [Ag 28 Cu 12 (SPhCl 2 ) 24 ] 1 (PPh 4 ) 4 , [Au x Ag 28- x Cu 12 (SPhCl 2 ) 24 ] 1 (PPh 4 ) 4 ( x = 1.32), [Au x Ag 28- x Cu 12 (SPhCl 2 ) 24 ] 1 (PPh 4 ) 3 ( x = 7.56), [Au x Ag 28- x Cu 12 (SPhCl 2 ) 24 ] 1 (PPh 4 ) 4 ( x = 7.76), [Au 12 Cu y Ag 32- y (SPhCl 2 ) 30 ] 4− and [Au 12 Ag 32 (SPhCl 2 ) 30 ] 1 [N(C 4 H 9 ) 4 ] 4 nanoclusters Single crystals of these nanoclusters were cultivated at room temperature by vapor diffusing the ethyl ether into the DMF solution of them. After 21 days, black crystals were collected, and the structures of these nanoclusters were determined. The CCDC number of [Ag 28 Cu 12 (SPhCl 2 ) 24 ] 1 (PPh 4 ) 4 is 2009375; the CCDC number of [Au x Ag 28- x Cu 12 (SPhCl 2 ) 24 ] 1 (PPh 4 ) 4 ( x = 1.32) is 2009456; the CCDC number of [Au x Ag 28- x Cu 12 (SPhCl 2 ) 24 ] 1 (PPh 4 ) 3 ( x = 7.56) is 2009457; the CCDC number of [Au x Ag 28- x Cu 12 (SPhCl 2 ) 24 ] 1 (PPh 4 ) 4 ( x = 7.76) is 2083130; the CCDC number of [Au 12 Cu y Ag 32- y (SPhCl 2 ) 30 ] 4− is 2009378; and the CCDC number of [Au 12 Ag 32 (SPhCl 2 ) 30 ] 1 [N(C 4 H 9 ) 4 ] 4 is 1936551. Of note, the perfect crystal data of [Au 12 Cu y Ag 32- y (SPhCl 2 ) 30 ] 4− remained unavailable despite our repeated efforts, and we only got its kernel structure (i.e., Au 12 Cu y Ag 32- y S 30 ) while the peripheral C, H, and Cl atoms were hard to determine. Co-crystallization between M 40 (SPhCl 2 ) 24 and M 44 (SPhCl 2 ) 30 nanoclusters ([Au 4 Ag 24 Cu 12 (SR) 24 ] 2 [Au 12 Cu y Ag 32- y (SR) 30 ] 1 , y = 3.74) In all, 20 mg of Au 12 Cu y Ag 32- y (SPhCl 2 ) 30 (8-min sample in Supplementary Fig. 8 ) and 20 mg of Au x Ag 28- x Cu 12 (SPhCl 2 ) 30 (2-min sample in Supplementary Fig. 14 ) were dissolved in 5 mL of DMF. Single crystals of the co-crystallized nanoclusters were cultivated at room temperature by vapor diffusing the ethyl ether into the DMF solution. After 21 days, black crystals were collected, and the structure of the co-crystallized nanoclusters was determined. The CCDC number of the co-crystallized [Au 4 Ag 24 Cu 12 (SR) 24 ] 2 [Au 12 Cu y Ag 32- y (SR) 30 ] 1 ( y = 3.74) is 2009377. Time-dependent ESI-MS of the Au alloying process on Ag 28 Cu 12 (SPhCl 2 ) 24 In total, 20 mg of Ag 28 Cu 12 (SPhCl 2 ) 24 was firstly dissolved in 20 mL of CH 2 Cl 2 and then 5 mg of Au(I)-SPhCl 2 complexes (powder) was added in. The ESI-MS measurement of the reaction was performed every minute. X-ray absorption fine structure spectroscopy measurements XAFS measurements at the Au L3-edge (11919 eV) were performed at the beamline BL14W1 station of the Shanghai Synchrotron Radiation Facility (SSRF), China. The storage ring of the SSRF was working at an energy of 3.5 GeV with an average electron current of 300 mA. The hard X-ray was monochromatized with a Si (311) monochromator. XAFS data were collected in the transmission mode in the energy range from 200 below to 1000 eV above the Au L3-edge. The acquired XAFS data were processed according to the standard procedures using the ARTEMIS module implemented in the IFEFFIT software packages. X-ray crystallography For the crystal date of Ag 28 Cu 12 (SPhCl 2 ) 24 , Au x Ag 28- x Cu 12 (SPhCl 2 ) 24 ( x = 1.32), Au 12 Cu y Ag 32- y (SPhCl 2 ) 30 , Au x Ag 28- x Cu 12 (SPhCl 2 ) 24 ( x = 7.76), and the co-crystallized [Au 4 Ag 24 Cu 12 (SR) 24 ] 2 [Au 12 Cu y Ag 32- y (SR) 30 ] 1 ( y = 3.74): the data collection for single-crystal X-ray diffraction was carried out on Stoe Stadivari diffractometer under nitrogen flow, using graphite-monochromatized Cu Kα radiation (λ = 1.54186 Å). For the crystal date of Au x Ag 28- x Cu 12 (SPhCl 2 ) 24 ( x = 7.56), Au 12 Ag 32 (SPhCl 2 ) 30 : the data collection for single crystal X-ray diffraction was carried out on a Bruker Smart APEX II CCD diffractometer under liquid nitrogen flow, using graphite-monochromatized Mo Kα radiation (λ = 0.71069 Å). Data reductions and absorption corrections were performed using the SAINT and SADABS programs, respectively [63] . The structure was solved by direct methods and refined with full-matrix least squares on F 2 using the SHELXTL software package [64] . All non-hydrogen atoms were refined anisotropically, and all the hydrogen atoms were set in geometrically calculated positions and refined isotropically using a riding model. All crystal structures were treated with PLATON SQUEEZE, and the diffuse electron densities from these residual solvent molecules were removed [65] . Characterization The UV-vis absorption spectra of nanoclusters were recorded using an Agilent 8453 diode array spectrometer. Electrospray ionization mass spectrometry (ESI-MS) measurements were performed by MicrOTOF-QIII high-resolution mass spectrometer. The sample was directly infused into the chamber at 5 μL/min. For preparing the ESI samples, nanoclusters were dissolved in CH 2 Cl 2 (1 mg/mL) and diluted ( v / v = 1:2) by CH 3 OH. Energy-dispersive X-ray spectroscopy (EDS) mapping of nanoclusters were characterized by SEM (Quanta 400 F). X-ray photoelectron spectroscopy (XPS) measurements were performed on a Thermo ESCALAB 250 configured with a monochromatized Al K α (1486.8 eV) 150 W X-ray source, 0.5 mm circular spot size, flood gun to counter charging effects, and analysis chamber base pressure lower than 1 × 10 −9 mbar.